Electronic transport and device prospects of monolayer molybdenum disulphide grown by chemical vapour deposition Layered transition metal dichalcogenides display a wide range of attractive physical and chemical properties and are potentially important for various device applications. Here we report the electronic transport and device properties of monolayer molybdenum disulphide grown by chemical vapour deposition. We show that these devices have the potential to suppress short channel effects and have high critical breakdown electric field. However, our study reveals that the electronic properties of these devices are at present severely limited by the presence of a significant amount of band tail trapping states. Through capacitance and ac conductance measurements, we systematically quantify the density-of-states and response time of these states. Because of the large amount of trapped charges, the measured effective mobility also leads to a large underestimation of the true band mobility and the potential of the material. Continual engineering efforts on improving the sample quality are needed for its potential applications. Two-dimensional materials are attracting considerable attention due to their unique electronic, optical and mechanical properties [1] . Following the success of graphene, a group of 2D materials known as the transition metal dichalcogenides (TMDs) has begun to garner attention. Among them, molybdenum disulphide (MoS 2 ) is probably one of the most explored TMDs [2] , [3] . The sizeable (1.8 eV) direct band gap of monolayer MoS 2 (ref. 4 ) makes it a potential material for not only digital electronics but also numerous photonic applications such as light emitter [5] , photodetectors [6] , [7] and solar cells [8] . Excellent mechanical flexibility of MoS 2 also makes it a compelling semiconducting material for flexible electronics [9] , [10] . Most existing studies and device demonstrations were performed on exfoliated MoS 2 flakes [11] , [12] , [13] , [14] , [15] , [16] , [17] , [18] , [19] . In particular, field-effect-transistors based on monolayer MoS 2 was found to exhibit high on/off ratios of ~10 8 , steep subthreshold swing of ~70 mV dec −1 (refs 18 , 20 ), with reported electron effective mobility ranging from 1 to 480 cm 2 V −1 s −1 (refs 14 , 17 , 20 , 21 , 22 , 23 , 24 , 25 , 26 ) depending on the device structures, dielectric environment and processing [21] , [27] . These encouraging early reports coupled with continual engineering efforts [28] present a compelling case for monolayer MoS 2 as an alternative to traditional organic material or amorphous silicon for low-end applications with basic requirement of an effective mobility of >30 cm 2 V −1 s −1 (ref. 20 ) for example, high resolution displays and photodetection [6] , [7] . Recently, the advent of mass production technologies has enabled scalable growth of polycrystalline monolayer MoS 2 by chemical vapour deposition (CVD) [29] , [30] , [31] , [32] , hence providing a commercially viable path towards MoS 2 electronics at low cost [33] . However, the mobility of CVD MoS 2 is typically much lower than its exfoliated counterpart, with reported values in the range of 5 to 22 cm 2 V −1 s −1 (refs 34 , 35 , 36 ). The physical origin of the differences between CVD and exfoliated MoS 2 is not clear at present; however, structural defects [37] such as vacancies, dislocations, grain boundaries as well as charged interfacial states due to the dielectrics in contact [14] can be responsible for the degradation in mobility. Although this problem has presented a major hurdle to the realization of wafer-scale MoS 2 electronics and photonics, systematic studies of it are very few [35] . Very recently, the MoS 2 community realized that there are technical difficulties to achieve accurate mobility extraction due to the role of contacts and fringing capacitive contributions [38] . Four-terminal Hall effect measurements are more accurate, but have only been demonstrated at very high carrier densities using an electrolyte gating scheme [26] or at very low temperatures [17] . These Hall measurements were all performed on exfoliated MoS 2 , and will be more challenging to perform in CVD samples due to significantly larger amount of localized states, as will be discussed in this manuscript. Here, we present a systematic methodology for characterizing electronic properties of scalable CVD MoS 2 , reporting also the presence of significant amounts of band tail states and their profound impact on the electrical device performance. The density distribution and dynamics of these trap states of CVD MoS 2 are characterized through systematic capacitance and ac conductance measurements. Extraction of basic electronic transport quantities like the mobility edge and effective mobility is performed using four-probe current measurements. Complementary modelling allows us to draw insights into relevant device quantities such as the fractional occupation of band and trap states, band mobility and the anomalous subthreshold slope. Lastly, high-field electrical behaviour such as drain-induced barrier lowering and critical breakdown fields are examined. Characterization of monolayer CVD MoS 2 Monolayer MoS 2 was synthesized by CVD, using solid sulphur (S) and molybdenum oxide (MoO 3 ) as the precursors and perylene-3,4,9,10-tetracarboxylic acid tetra-potassium salt (PTAS) [39] as the seed for the CVD growth (see Methods for details). Hall-bar devices were fabricated on these CVD MoS 2 monolayers. 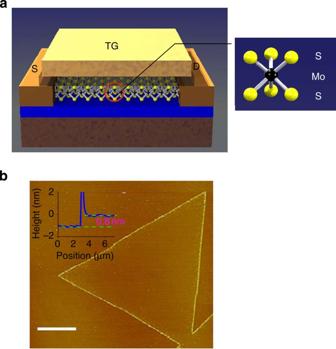Figure 1: Molybdenum disulphide physical properties and device structure. (a) Schematic of MOSFET with monolayer chemical vapour deposition (CVD) grown molybdenum disulphide (MoS2). (b) AFM image of CVD grown MoS2on SiO2/Si substrate. The scale bar in the AFM image is 10 μm. The inset shows the step height profile of MoS2in the AFM image. Figure 1a illustrated the schematic of the device. The top gate dielectrics are 2 nm aluminium deposited by e-beam evaporation and re-oxidized as a seed layer, followed by 30 nm HfO 2 deposited by atomic layer deposition (ALD). The details of the device process are discussed in Methods. The atomic force microscopy (AFM) image and the step height profile at the boundary of a MoS 2 triangular area are shown in Fig. 1b and the inset of Fig. 1b , respectively. The thickness of the MoS 2 layer is measured to be about 0.8 nm, confirming its monolayer character. The Raman spectrum of the CVD MoS 2 is shown in Supplementary Fig. 1 . The E 2g and A 1g modes are at around 383 and 403 cm −1 , respectively. Comparing the peak position with the spectrum obtained from the exfoliated monolayer MoS 2 (ref. 40 ), we further verify that the MoS 2 film is monolayer. Figure 1: Molybdenum disulphide physical properties and device structure. ( a ) Schematic of MOSFET with monolayer chemical vapour deposition (CVD) grown molybdenum disulphide (MoS 2 ). ( b ) AFM image of CVD grown MoS 2 on SiO 2 /Si substrate. The scale bar in the AFM image is 10 μm. The inset shows the step height profile of MoS 2 in the AFM image. Full size image Density and dynamics of band tail states At present, the reported values of the electron mobility in CVD-grown MoS 2 devices [34] , [35] , [36] are at least two orders of magnitude smaller than the intrinsic limit [41] , suggesting a high degree of disorder and scattering. An inhomogeneous potential distribution in a semiconductor leads to the smearing of the band edge and the formation of a tail of band gap state [42] . For example, this inhomogeneity could be the result of a random distribution of trapped charges in sulphur vacancies in MoS 2 itself [43] or at MoS 2 –dielectric (SiO 2 or high-k dielectric) interfaces [14] . Structural defects [37] , for example, simple vacancies [43] , dislocations and grain boundaries, would also lead to localized gap states. The electronic states in the band tail can be characterized using standard capacitance and ac conductance measurement commonly used in the study of semiconductor devices [44] . Here, these localized states respond like traps with different time constants τ it and are electrically equivalent to an additional capacitance and resistance in parallel to the semiconductor capacitance. The gate-to-channel capacitance and resistance were measured on the Hall-bars, with high terminal on the top gate and low terminal on the source, drain and all four voltage probing leads simultaneously, as shown in Supplementary Fig. 2 . The measured capacitance as a function of frequency is shown in Fig. 2a . The observed double hump feature indicates at least two types of traps with different time constants at a given gate voltage. Herein, we denote these traps by the labels ‘M’ and ‘B’, for reasons that will be made apparent below. The equivalent circuit model of the device is shown in Fig. 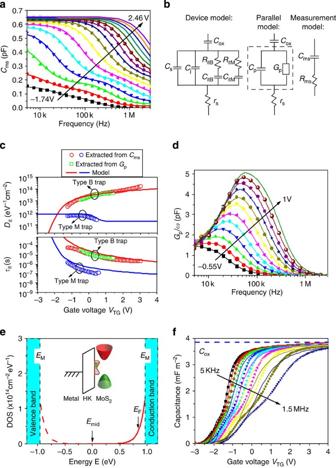Figure 2: Characterization of the density and dynamics of band tail states. (a) Capacitance as a function of frequency measured at various gate voltages. The device width is 4 μm and length is 44 μm. The symbols are the experimental results and the lines are fittings using the device model shown in (b). (b) The equivalent circuit model of the device, simplified parallel model and the measurement model in series mode. (c) Density and time constant of trap states as a function of gate voltages. The symbols are experimental results extracted from the capacitanceCmsand ac conductanceGp. The lines are models, see text. (d) Extracted ac conductance over angular frequencyGp/ωas a function of frequencyfat various gate voltages. (e) Parameterized model,Dn(E), describing the electronic density-of-states of both the extended and localized states. The valence density-of-state is also included in the illustration using the mirror image of conduction density-of-state. The inset illustrates the band diagram of MoS2MOSFET. (f) Multi-frequency capacitance of MoS2Hall-bar as a function of gate voltage. The symbols are experimental results and the lines are the modelling results. 2b with total impedance given by: Figure 2: Characterization of the density and dynamics of band tail states. ( a ) Capacitance as a function of frequency measured at various gate voltages. The device width is 4 μm and length is 44 μm. The symbols are the experimental results and the lines are fittings using the device model shown in ( b ). ( b ) The equivalent circuit model of the device, simplified parallel model and the measurement model in series mode. ( c ) Density and time constant of trap states as a function of gate voltages. The symbols are experimental results extracted from the capacitance C ms and ac conductance G p . The lines are models, see text. ( d ) Extracted ac conductance over angular frequency G p / ω as a function of frequency f at various gate voltages. ( e ) Parameterized model, D n ( E ), describing the electronic density-of-states of both the extended and localized states. The valence density-of-state is also included in the illustration using the mirror image of conduction density-of-state. The inset illustrates the band diagram of MoS 2 MOSFET. ( f ) Multi-frequency capacitance of MoS 2 Hall-bar as a function of gate voltage. The symbols are experimental results and the lines are the modelling results. Full size image where ω is the angular frequency, C s is the quantum capacitance of the MoS 2 , C j is the parasitic capacitance, C ox is the oxide capacitance, r s is the series resistance, Y itM and Y itB are the traps’ admittance. Here Y itB =[ τ itB / C itB +1/( iωC itB )] −1 , where C itB and τ itB are the capacitance and time constant of trap B. The trap capacitance C itB is related to the trap density D itB via the following: C itB = eD itB , where e is the elementary electric charge. Similar expressions apply to trap M. The measured capacitance in series mode C ms is related to the imaginary part of the total impedance Z by the following formula: The lines in Fig. 2a are the fits using this model. We can see that the model provides an excellent fit to the experimental data. From the fitting, we can extract the density of traps and their time constant as a function of gate voltage, shown in Fig. 2c . Here, we observe that traps ‘M’ and ‘B’ are populated predominately within the ‘mid-gap’ and ‘band edge’ regions, respectively. Alternatively, the density and time constant of the traps can be extracted from the ac conductance G p (ref. 44 ). The ac conductance is obtained from the measured capacitance and resistance. The measured resistances as a function of gate voltage at various frequencies are shown in Supplementary Fig. 3 . The extraction method of ac conductance are described in more detail in the Supplementary Note 1 . The extracted ac conductance over angular frequency G p / ω is plotted as function of the driving frequencies f in Fig. 2d . Since the density-of-states of type B traps is several orders of magnitude larger than that of type M in this gate bias range, we expect the former to dominate the ac conductance. The relation between G p ( ω ) and the trap density D itB is given as the following (ref. 44 ): from which one can deduce the D itB and the respective time constant τ itB from the following simple relations [44] : Here, ( G p / ω ) peak is the maximum G p ( ω )/ ω value and f 0 is the frequency at which this maximum is obtained. Repeating the above procedure for different top gate voltages V TG allows us to extract D itB ( V TG ) and τ itB ( V TG ) as shown in Fig. 2c . From Fig. 2c , we see that the density-of-states and time constant of B type traps extracted based on the capacitance and ac conductance are in good agreement. Below, we present parameterized models for the electronic density-of-states and their time constants fitted to the experiments. We describe the electronic density-of-states of the measured distributed trap states at the band edge (that is, type B) and the extended states with two piece-wise functions as follows: and illustrate them in Fig. 2c,e . Here, D 0 is the 2D density-of-states for perfect crystalline MoS 2 , taken to be 3.3 × 10 14 eV −1 cm −2 , consistent with an effective mass of 0.4 m 0 at the conduction band minimum at the K valley for monolayer MoS 2 (ref. 45 ). Here we ignored contribution from the satellite valley along ΓK with energy 200 meV higher than the conduction band minimum [41] , [46] because the carrier population is insignificant at these energies at our biasing range. Furthermore, our MoS 2 devices are typically n-type doped. ϕ is the characteristic energy width of the band tail. In the limit of ϕ =0, D n ( E ) becomes a step function as required for perfect 2D crystals with the conduction band edge situated at E D . ϕ ′ is chosen so that the two piece-wise functions have continuous gradients at E D . Solving the electrostatics problem, to be described below, a best-fit to the experimentally extracted density-of-states yields the parameter set: α =0.33 and ϕ =100 meV. The comparison between the model D n ( V TG ) and the measured band tail states D itB ( V TG ) is shown in Fig. 2c , and the mid-gap states D itM ( V TG ) is described by an error function instead. The traps’ response time is fitted to an exponential model, and the comparison with experimental data is shown in Fig. 2c . With the parameterized density-of-states model, we can calculate the ac capacitance and compare against experiments. The Poisson equation describing the electrostatics of the problem can be expressed as: where t top is the ‘effective-oxide-thickness’ for the top gate dielectric, ε ox is the dielectric constant of silicon oxide, Q 0 is a constant that includes contributions from the fixed charges and doping in as-prepared MoS 2 and so on, and Q n is the electronic charges in the smeared out conduction band and can be computed from Q n = e ( E ) f n ( E , E F )d E where f n is the Fermi Dirac function. In solving for the self-consistent electrostatics described by using equation 8, the Fermi energy E F is taken to be the reference that is, E F =0. Once the electrostatics is determined, the admittance associated with each of the traps can then be computed via the following: and the total capacitance can be computed employing the equivalent circuit model in Fig. 2b and using equations (1) and (2). Reasonable agreement with the measured ac capacitance is obtained as shown in Fig. 2f . To summarize, the electronic density-of-states model described above is well-calibrated to the experimentally measured density and dynamics of the band tail states. It follows an exponentially decaying behaviour, with a significantly large energy width of ϕ =100 meV, suggesting a high degree of potential disorder and scattering. This model will be employed in the subsequent discussion to obtain other quantities of interest, such as the band mobility. Mobility edge The concept of a ‘mobility edge’ has greatly facilitated our understanding of electronic transport in a disordered system [47] . The mobility edge is a boundary located in the band tail, in which states above it are extended states with band transport, while those below it are localized states that conduct via thermally assisted mechanisms such as Mott variable range hopping (VRH) [48] , [49] , [50] or an Arrhenius-type activated behaviour [51] . Four-point variable temperature measurements were performed on our devices from 4.4 to 400 K as shown in Fig. 3a . We found that neither the VRH nor the Arrhenius model can individually describe the data satisfactorily over the whole temperature range. It is very likely that a combination of both transport mechanisms might be operating here. For example, the VRH usually dominates for localized states deep in the band tail, while the Arrhenius-type activated behaviour is more likely for shallow localized states. 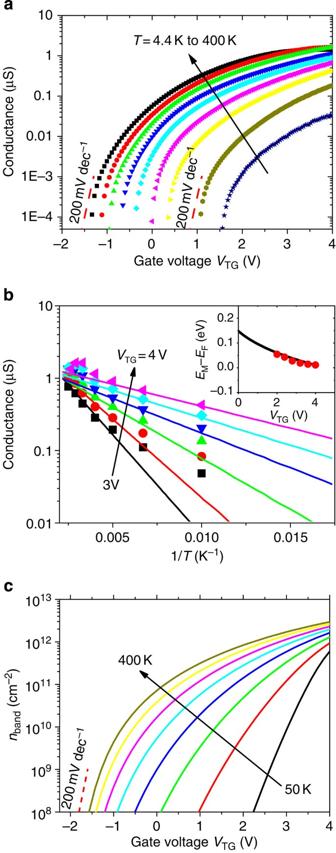Figure 3: Temperature dependence of conductance and activation energy. (a) Four-point conductance as a function of gate voltage measured at various temperatures from 4.4 to 400 K on a MoS2Hall-bar. (b) Conductance as a function of reverse of temperature 1/Tat various gate voltages. The inset shows the activation energy at various gate voltages fitted to the Arrhenius-activated energy model. The symbols are experimental results extracted from the conductance; the solid line gives the modeling results. (c) The calculated band carriers as a function of gate voltage at various temperatures. Figure 3: Temperature dependence of conductance and activation energy. ( a ) Four-point conductance as a function of gate voltage measured at various temperatures from 4.4 to 400 K on a MoS 2 Hall-bar. ( b ) Conductance as a function of reverse of temperature 1/ T at various gate voltages. The inset shows the activation energy at various gate voltages fitted to the Arrhenius-activated energy model. The symbols are experimental results extracted from the conductance; the solid line gives the modeling results. ( c ) The calculated band carriers as a function of gate voltage at various temperatures. Full size image The conductance versus the inverse of temperature (1/ T ) is shown in Fig. 3b , showing the exponential decrease with 1/ T over the intermediate temperature range, where the conductance G can be described by: where E a is the activation energy, k B is the Boltzmann constant and G 0 is a fitting parameter. This allows us to extract the activation energy E a = E M − E F . The measured E a (versus V TG ) is compared with the model (see Fig. 3c inset), which allows us to determine the location of the mobility edge in the energy band picture. We found that in our devices E M is ≈0.01 eV above E D , as illustrated in Fig. 2e . We also noticed a departure from activated behaviour at lower temperature or bias, indicating the possible onset of an additional transport mechanism such as VRH. The extracted activation energy in the inset of Fig. 3b suggests that, in most of our gate biases, the Fermi level does not exceed the mobility edge energy. However, at large V TG that is, V TG >2 V , the Fermi energy is within tens of meV from the mobility edge. Hence, one can expect an appreciable fraction of extended states occupation due to thermal smearing. The calculated band carrier densities as a function of gate voltage at various temperatures are shown in Fig. 3c . Transport coefficients The ‘effective mobility’, or sometimes referred to as the ‘drift mobility’, is a commonly used transport coefficient in semiconductors [52] . It is defined as the ratio of the measured conductivity to the total charge density that is, μ eff = σ / Q total . The total charge density Q total is typically estimated from C ox ( V g − V T ), where C ox is the oxide capacitance, V g is the gate voltage and V T is the threshold voltage. We extract C ox from the measured capacitance at strong accumulation. 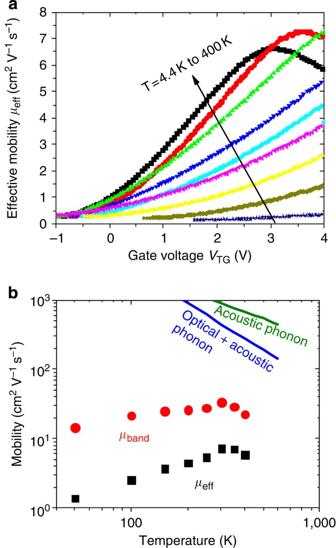Figure 4: Effective mobility and band mobility. (a) Effective mobility as a function of gate voltage measured at various temperatures in MoS2Hall-bar. (b) Effective mobility and the corresponding band mobility as a function of temperature atVTG=4V. The mobility limited by MoS2phonons scattering based on theoretical calculations41are also plotted for comparison. Figure 4a shows the effective mobility as a function of gate voltage at different temperatures. The effective mobility is <10 cm 2 V −1 s −1 over the range of temperature and applied bias in our experiments. Contact resistance is eliminated in our measurement that employs a four-probe scheme. The measured effective mobility is significantly lower than the phonon-limited intrinsic mobility in monolayer MoS 2 , predicted to be over 400 cm 2 V −1 s −1 (ref. 41 ), and the highest measured mobility of ~200 cm 2 V −1 s −1 in exfoliated MoS 2 devices [20] . However, it is consistent with results on similar CVD-grown MoS 2 devices that report mobilities in the range of 5 to 25 cm 2 V −1 s −1 (ref. 35 ). The significantly lower mobility for CVD-grown MoS 2 is, to a large part, due to the presence of traps. Figure 4: Effective mobility and band mobility. ( a ) Effective mobility as a function of gate voltage measured at various temperatures in MoS 2 Hall-bar. ( b ) Effective mobility and the corresponding band mobility as a function of temperature at V TG =4V. The mobility limited by MoS 2 phonons scattering based on theoretical calculations [41] are also plotted for comparison. Full size image The total charge density includes both the free and trapped charges: Q total = e ( n loc + n band ) where n loc and n band refer to the density of occupied states below and above the mobility edge, respectively. Another commonly used transport coefficient in a disordered system is the ‘band mobility’ [53] , [54] . It is defined as the ratio of the measured conductivity to the density of occupied states above the mobility edge (that is, extended states): In general, the density of the extended states is difficult to measure, since the large amount of localized states would result in large noise-to-signal ratio the in the Hall measurement. Up to now, the Hall effect has only been observed in exfoliated MoS 2 with very high carrier density induced by an electrolyte gating scheme [26] or at very low temperatures [17] . Previously, we obtained D n ( E ) in conjunction with E M in the energy band picture. Solving the electrostatics in conjunction with the above information would allow us to estimate the fraction of localized and extended states. Figure 3c plots the computed n band ( V TG ) at different temperatures. The result indicates that n band only accounts for <25% of n total . Only at high temperature or bias, n band can exceed 25% that is, T >300 K and V TG >2V. The comparison between the extracted band mobility and measured effective mobility is shown in Fig. 4b . The band mobility is several times higher than the effective mobility, but still significantly lower than the phonon-limited mobility as predicted in ref. 41 . This mobility degradation may involve many sources of scattering. For example, structural defects in CVD MoS 2 layer and grain boundaries can induce short-range scattering. Surface polar phonon either in the high-k dielectrics (HfO 2 and AlO x ) or in the SiO 2 substrate underneath can also play a role. However, the significant trap population measured here suggests that Coulomb scattering due to trapped charges is the likely limiting factor for the electron mobility. Because of the parabolic band structure of MoS 2 , the energy averaged scattering time due to Coulomb scattering should increase proportionally to temperature [55] μ k B T . This is also consistent with the observed trend in Fig. 4b for temperature below 300 K. Above this temperature phonon scattering takes over. Subthreshold swing In an ideal semiconductor, the subthreshold swing is given by [52] : S = k B T In(10)(1+ C D / C ox ), where C D is the depletion capacitance. The subthreshold swing increases linearly with temperature, since the carrier density increases exponentially with temperature n exp . In our device, we observed that the subthreshold swing is ≈200 mV dec −1 and nearly independent of temperature, as shown in Fig. 3a . Similar observations were made on MoS 2 flakes [11] . This departure from the ideal behaviour can be understood by recalling that the band tail is distributed in energy, that is, exp , with an energy width that is significantly larger than the thermal energy that is, φ >> k B T . Indeed, the calculated subthreshold behaviour confirms that temperature does not have a significant effect, as shown in Fig. 3c . Hence, the observed temperature-independent subthreshold swing reinforced our earlier conclusions on the existence of band tail states. Drain-induced barrier lowering The electrostatic integrity of an electronic device upon downscaling is often quantified by evaluating the amount of drain-induced barrier lowering (DIBL) [56] . This measures the reduction in threshold voltage due to the applied drain bias. A common approach used to suppress DIBL involves reducing the channel thickness, since the minimum channel length needed to preserve the long channel behaviour is typically ~4–5 times the electrostatic scaling length λ = for a planar device structure [57] , [58] , where ε s and ε ox are the dielectric constants of the semiconductor and the gate oxide, and t s and t ox are the thicknesses of the semiconductor and gate oxide, respectively. In this regard, thinner silicon has been pursued by using SOI (silicon-on-insulator) and ETSOI (extremely thin silicon-on-insulator). However, the mobility degrades markedly as the thickness is scaled down due to surface roughness [59] , [60] . Atomically thin 2D semiconducting material such as MoS 2 and WSe 2 are promising candidates in this regard. The typical DC performances of MoS 2 MOSFETs with various channel lengths are shown in Supplementary Fig. 4 . 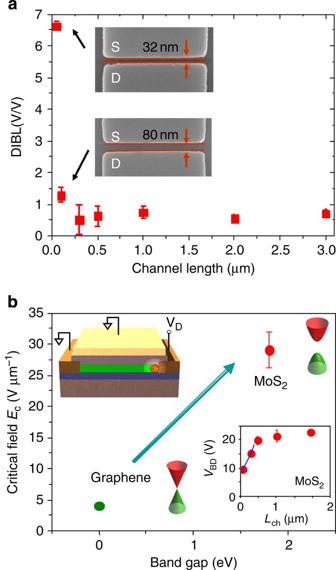Figure 5: Device properties at high electrical fields. (a) Drain-induced barrier lowering (DIBL) of MOSFET with CVD MoS2at various channel lengths. The inset shows the SEM image of the 32 and 80 nm channel length devices. (b) Critical electric field of CVD MoS2and graphene. The upper inset shows the measurement configuration. The lower inset shows the lateral breakdown voltage as a function of channel length for MOSFET with CVD MoS2. Figure 5a shows the DIBL of CVD MoS 2 MOSFET with variable channel lengths from 4 μm to 32 nm. Despite the thick dielectric used in our MOSFETs, (~34 nm HfO 2 / AlO x stack for the long channel devices, ~60 nm HfO 2 / AlO x for the short channel devices, limited by the bulging of gate dielectrics on the source/drain side wall), a clear upturn of DIBL is only observed at a channel length of 32 nm. Extrapolating to a device with a 3 nm HfO 2 gate insulator would predict a limiting channel length feature of ~7 nm. Theoretically, for a MOSFET with monolayer MoS 2 (channel thickness: ~0.8 nm, dielectric constant: 6.8~7.1 ε 0 , where ε 0 is the vacuum permittivity [61] ) and 1 nm equivalent oxide thickness (EOT), the electrostatic scaling length λ is only about 1.2 nm. These considerations suggest that MoS 2 could be a very promising material for scaled, high-density electronics. Figure 5: Device properties at high electrical fields. ( a ) Drain-induced barrier lowering (DIBL) of MOSFET with CVD MoS 2 at various channel lengths. The inset shows the SEM image of the 32 and 80 nm channel length devices. ( b ) Critical electric field of CVD MoS 2 and graphene. The upper inset shows the measurement configuration. The lower inset shows the lateral breakdown voltage as a function of channel length for MOSFET with CVD MoS 2 . Full size image Breakdown electric fields The large band gap of MoS 2 implies the possibility of device operation at higher voltages or electric fields. Figure 5b shows the critical breakdown fields of graphene and CVD MoS 2 MOSFETs devices. The measurement setup is shown on the upper-left inset of Fig. 5b . The channel-length dependence of breakdown voltage of MoS 2 MOSFETs is shown in the lower-right inset of Fig. 5b . The critical field can be extracted from the slope of the breakdown voltage versus channel length. Here we extracted the breakdown field from MoS 2 transistors with channel lengths of 80 and 285 nm. (More details about the breakdown test results of MoS 2 transistors and graphene transistors are shown in the Supplementary Figs 5 and 6 , and Supplementary Notes 2 and 3 .) The measured breakdown field of CVD MoS 2 is about five times larger than that of graphene and significantly larger than that of SOI with 100 nm silicon thickness [62] . In this regard, MoS 2 can also be a very promising platform for power devices. We have systematically studied the electronic transport properties of CVD MoS 2 devices. We report the observation of a significant amount of electronic trap states through capacitance and ac conductance measurements and their impact on the low-field electronic properties of MoS 2 devices. In particular, the measured effective mobility significantly underestimates the band mobility. An anomalous subthreshold behaviour, with distinctive temperature insensitivity, is also accounted for by the presence of these band tail states. We also studied the high-field electronic properties of MoS 2 devices and demonstrated the possibility to aggressively scale them down and their high breakdown electric fields. These attractive device attributes present a compelling case for wafer-scale monolayer MoS 2 as alternative to organic and other thin film materials for flexible electronics and photonics, including high resolution displays, photo-detection, logic electronics, power devices with solar energy collecting and so on. From the fundamental material stand point, understanding of the microscopic origin of these band tail states is critical for further improvement of the material’s electronic properties. Fabrication Large-scale monolayer MoS 2 was synthesized at 650 C by APCVD using perylene-3,4,9,10-tetracarboxylic acid tetra-potassium salt (PTAS) as the seed on SiO 2 /Si substrate [39] . Sulphur powder and molybdenum oxide (MoO 3 ) were used as the precursors for the synthesis. The SiO 2 thickness was 300 nm. In the Hall-bar and transistor devices, the source/drain contact metal stack consisted of Ti/Au/Ti (5/15/5 nm). The MoS 2 channel was patterned using electron beam lithography and oxygen plasma etching. The top gate dielectric comprised an AlO x /HfO 2 stack. The AlO x was formed by electron beam evaporation of 2 nm of aluminum metal followed by its natural oxidization in air for a few hours. The 30 nm thick HfO 2 layer was formed using atomic layer deposition (ALD) at 170 degrees. The top gate electrode was Ti/Au (5/40 nm). Characterization The capacitances were measured using Agilent B1500 Semiconductor Device Analyzer produced by Agilent technology. The temperature dependence of conductance was measured using cryogenic probestation produced in Lake Shore Cryotronics, Inc. The Raman spectrum was taken using Labram Aramis produced by Horiba Jobin Yvon. Scanning electron microscopy was measured using Leo 1560 produced by Carl Zeiss. How to cite this article: Zhu, W. et al. Electronic transport and device prospects of monolayer molybdenum disulphide grown by chemical vapour deposition. Nat. Commun. 5:3087 doi: 10.1038/ncomms4087 (2014).